Giant nonlinear optical activity in two-dimensional palladium diselenide 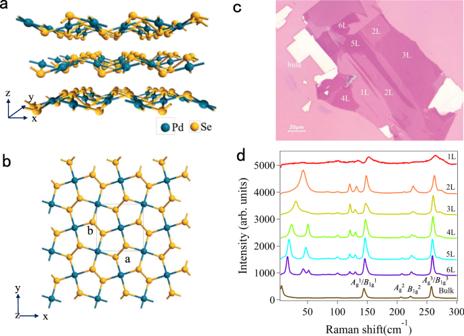Fig. 1: Crystallographic structure and optical characteristics of a few-layer PdSe2. aThe lattice structure of PdSe2flakes with a puckered pentagonal. The unit cell vectors are denoted by the x, y, and z. Blue and yellow globes denote the Pd and Se atoms, respectively.bTop view of the atomic crystal structure of monolayer PdSe2. The black dotted frame represents a unit cell of PdSe2. Theaandbdenote the lattice constants along the x and y directions, respectively.cThe optical microscope image of a few-layer PdSe2on the silicon substrate with a 285 nm SiO2layer. The numbers of sample layers containing 1–6 L were marked with white letters, and the scale bar is 20  μm.dRaman spectra of the 1–6 L and bulk PdSe2flakes with the same intensity axis. The low-frequency Raman peaks (0−100 cm−1) were robust and even exceeded that of the high-frequency modes. The Raman vibration modes of bulk PdSe2were marked asAg1,Ag2,Ag3,B1g1,B1g2, andB1g3mode. Nonlinear optical effects in layered two-dimensional transition metal chalcogenides have been extensively explored recently because of the promising prospect of the nonlinear optical effects for various optoelectronic applications. However, these materials possess sizable bandgaps ranging from visible to ultraviolet region, so the investigation of narrow-bandgap materials remains deficient. Here, we report our comprehensive study on the nonlinear optical processes in palladium diselenide (PdSe 2 ) that has a near-infrared bandgap. Interestingly, this material exhibits a unique thickness-dependent second harmonic generation feature, which is in contrast to other transition metal chalcogenides. Furthermore, the two-photon absorption coefficients of 1–3 layer PdSe 2 ( β ~ 4.16 × 10 5 , 2.58 × 10 5 , and 1.51 × 10 5 cm GW −1 ) are larger by two and three orders of magnitude than that of the conventional two-dimensional materials, and giant modulation depths ( α s ~ 32%, 27%, and 24%) were obtained in 1–3 layer PdSe 2 . Such unique nonlinear optical characteristics make PdSe 2 a potential candidate for technological innovations in nonlinear optoelectronic devices. Nonlinear optical (NLO) properties play an increasingly significant role in the development of laser technology, optical spectroscopy, and material structure analysis methodologies [1] , [2] , [3] , [4] . Recently, the study of NLO activity in two-dimensional (2D) layered materials (such as graphene, transition metal chalcogenides (TMDCs), and black phosphorus (BP)) has made significant progress [5] , [6] , [7] , [8] , [9] , [10] , [11] , [12] . The extraordinary nonlinearities of graphene, including saturable absorption (SA) [13] , [14] , optical limiting [15] and harmonic generation [16] , have attracted great interest. However, the inherent properties of graphene, like its zero-bandgap and centrosymmetric crystal structure [17] , hinder the study of its NLO effects, including the second harmonic generation (SHG) and multiphoton absorption features. On the contrary, BP possesses intrinsic anisotropy, strong light-matter interaction, layer-dependent direct bandgap (0.3–2 eV), and a wide range of adjustable optical response [18] , [19] , leading to high SA modulation depths (~27.6% at 400 nm, ~12.4% at 800 nm [20] ) and a large two photon absorption (TPA) coefficient ((−6.98 ± 0.6) × 10 3 cm GW −1 [21] ). However, BP lacks sufficient air stability, resulting in the rapid degradation of its NLO properties. Meanwhile, the most studied TMDC materials (MX 2 , M = Mo, W, and X = S, Se, Te) that exhibit various fascinating NLO activities, such as SHG, SA and TPA, have sizable bandgaps ranging from visible to the ultraviolet region (1–2.5 eV) and there is a shortage of narrow-bandgap materials [22] . Interestingly, PdSe 2 is a pentagonal 2D material with robust anisotropy, high carrier mobility, and air stability, that give it considerable advantages in nonlinear optoelectronic devices [23] . In addition, PdSe 2 has a modifiable thickness-dependent bandgap from 0.03 to 1.37 eV [24] , filling the interspace between zero-gap graphene and large-gap TMDCs. Meanwhile, Xu et al. demonstrated the ultrafast SA performance of liquid-phase exfoliated PdSe 2 that generated the dissipative soliton and pulse energy [25] . Zhang et al. experimentally investigated the mode-locked Er and Yb-doped operations in multilayer PdSe 2 [26] . These works demonstrate the capacity of PdSe 2 for broadband ultrafast photonic devices. However, to date, the current experimental investigation of the NLO activities of PdSe 2 (especially the monolayer sample) is insufficient. Therefore, an extensive and in-depth study of the NLO behavior of PdSe 2 is of great significance for the expansion of its optoelectronic applications. Herein, we report the fabrication of large-size PdSe 2 flakes with different layers and present a comprehensive investigation of thickness-dependent NLO properties of the PdSe 2 flakes. Extraordinarily, owing to its unique layer-dependent inversion symmetry, PdSe 2 exhibits a SHG behavior that is totally opposed to that in other 2D materials [27] , [28] . Moreover, the PdSe 2 flakes exhibit giant TPA coefficients ( β ) that are two to three orders of magnitude larger compared to that of the conventional semiconductors [29] , [30] , [31] . Importantly, excellent saturable absorption was observed in 1–3 layer (L) PdSe 2 , with much higher modulation depths ( α s ) than that of the most other 2D materials [32] , [33] , [34] . These findings not only provide profound insights into the NLO features of this innovative nanomaterial, but also open an avenue for future nonlinear optoelectronic applications. Crystal structure and characterization of few-layer PdSe 2 flakes The unique optical characteristics of PdSe 2 are correlated to its special structure. It has a stratiform structure that is identical to some of the other 2D materials (graphene, hexagonal boron nitride (hBN), BP, and TMDCs), as shown in Fig. 1a . The Pd and Se atoms combine to form a covalent bond within a monolayer, and the van der Waals (vdWs) force dominates the interactions between adjacent layers. In the side view, PdSe 2 exhibits a unique plicate crystal structure with a monolayer vertical plicate height of 1.604 Å. In comparison to the traditional 2D materials with the highly symmetric hexagonal honeycomb structure, the Pd and Se atoms in PdSe 2 constitute an asymmetric pentagonal structure (Fig. 1b ). The ultrathin PdSe 2 crystal displays robust interlayer coupling with a relatively large binding energy of 190 meV/atom [35] , as manifested in the process of mechanical exfoliation. Monolayer and few-layer PdSe 2 flakes are difficult to be obtained by the conventional scotch tape method [23] , [36] . Instead, the gold-assisted exfoliation method was adopted to acquire the large-size monolayer and few-layer PdSe 2, as shown in Fig. 1c on the Si/SiO 2 substrates. The height profiles of the PdSe 2 samples were obtained by atomic force microscopy (AFM) measurements (Fig. S1 in Supplementary Information). According to the measurements, the average thickness of a single layer PdSe 2 is 0.7 nm. Recently, Raman technology has been demonstrated as an excellent approach in determining the layer number of various 2D materials [37] , [38] , [39] , [40] . Through analyzing the Raman spectrum, the layer number of a thin sample can be identified quickly, precisely and non-destructively. The Raman spectra of the 1–6 L and bulk PdSe 2 samples at a wavenumber range of 0–300 cm −1 were obtained to estimate the layer numbers (Fig. 1d ). Obviously, the Raman peak position varied gradually as the layer number increased. It is worth mentioning that the Raman peaks in the low-frequency region (0–100 cm −1 ) varied by a large margin. The low-frequency Raman modes indicate the occurrence of interlayer vibrations in the samples that were robust, and even exceeded those of the high-frequency modes (100–300 cm −1 ), which were attributed to the strong interlayer coupling of PdSe 2 . The peak positions of the low-frequency Raman modes have a specific relationship with the layer numbers, as shown in Fig. S2 in Supplementary Information. Because of the significant shifts of the low-frequency Raman modes, the layer number could be determined precisely. The feasibility and specific operation of such approach have been reported in detail in our previous work [24] . Fig. 1: Crystallographic structure and optical characteristics of a few-layer PdSe 2 . a The lattice structure of PdSe 2 flakes with a puckered pentagonal. The unit cell vectors are denoted by the x, y, and z. Blue and yellow globes denote the Pd and Se atoms, respectively. b Top view of the atomic crystal structure of monolayer PdSe 2 . The black dotted frame represents a unit cell of PdSe 2 . The a and b denote the lattice constants along the x and y directions, respectively. c The optical microscope image of a few-layer PdSe 2 on the silicon substrate with a 285 nm SiO 2 layer. The numbers of sample layers containing 1–6 L were marked with white letters, and the scale bar is 20  μm. d Raman spectra of the 1–6 L and bulk PdSe 2 flakes with the same intensity axis. The low-frequency Raman peaks (0−100 cm −1 ) were robust and even exceeded that of the high-frequency modes. The Raman vibration modes of bulk PdSe 2 were marked as A g 1 , A g 2 , A g 3 , B 1g 1 , B 1g 2 , and B 1g 3 mode. Full size image Furthermore, the high-resolution transmission electron microscopy (HRTEM) characterization was performed to reveal the atomic structure of PdSe 2 . The periodic atomic arrangement of PdSe 2 could be distinctly observed, and the sample had a flat surface (Fig. 2a ). No obvious defects were observed, indicating high crystallinity of the samples. 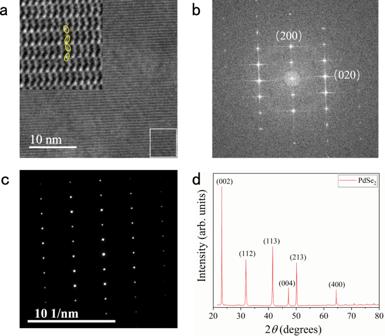Fig. 2: TEM and XRD characterizations of PdSe2flakes. aHRTEM image of the few-layer region of PdSe2flakes. The inset shows a zoom-in of the white square regions, revealing the atomic models. The scale is marked in the lower-left corner.bFFT diffraction patterns of the solid white areas highlighted on the image (a).cSAED pattern of the PdSe2.dXRD pattern of bulk PdSe2is in good agreement with the standard PDF card (PDF#97-017-0327). The diffraction pattern exhibits six robust peaks at 23.1, 31.8, 41.5, 47.2, 50.14, and 64.4°, respectively. Figure 2b shows the fast Fourier transform (FFT) diffraction patterns. The distinct diffraction spots correspond to the two principle crystal planes of (200) and (020). The selected-area electron diffraction (SAED) pattern was taken from the few-layer region of PdSe 2 (Fig. 2c ), indicating the high-quality single-crystal structure and confirming the isometric system of PdSe 2 . For the further investigation of our experimentally prepared PdSe 2 , X-ray diffraction (XRD) characterization was performed. As shown in Fig. 2d , the diffraction pattern exhibits six robust peaks at 23.1, 31.8, 41.5, 47.2, 50.14, and 64.4°, corresponding to (002), (112), (113), (004), (213), and (400) atomic planes of PdSe 2 , demonstrateing the high crystal quality of the sample [41] . Fig. 2: TEM and XRD characterizations of PdSe 2 flakes. a HRTEM image of the few-layer region of PdSe 2 flakes. The inset shows a zoom-in of the white square regions, revealing the atomic models. The scale is marked in the lower-left corner. b FFT diffraction patterns of the solid white areas highlighted on the image ( a ). c SAED pattern of the PdSe 2 . d XRD pattern of bulk PdSe 2 is in good agreement with the standard PDF card (PDF#97-017-0327). The diffraction pattern exhibits six robust peaks at 23.1, 31.8, 41.5, 47.2, 50.14, and 64.4°, respectively. Full size image SHG properties of PdSe 2 flakes To better understand the NLO characteristics of the PdSe 2 flakes, the SHG properties of few-layer PdSe 2 at the excitation wavelength of 800 nm were studied in detail. For the monolayer region, the detected SHG signal was negligible. When the laser spot was switched to the bilayer area, strong signals could be observed at 400 nm. In order to further demonstrate the SHG signal dependence on the PdSe 2 layer number, the spatial mapping was implemented. The red box in Fig. 3a indicates the scanning regions of the sample, containing 1–5 L, 8 L, and bulk PdSe 2 flakes. Clearly, the SHG signals from even-numbered layers of PdSe 2 were strong, while the signals from odd-numbered layers and the bulk PdSe 2 were almost negligible (Fig. 3b ). In order to ensure sufficient sampling, spatial scanning of another sample (consisting of 1–7 L and bulk PdSe 2 ) was carried out and the same results were obtained, as can be seen in Fig. 3c, d . Such characteristics are exactly opposite to the SHG phenomenon displayed by other group VI 2D materials, where a strong SHG signal was only observed from the odd-numbered layers, and no signal was detected from even-numbered layers [27] , [28] , [42] . It is well known that strong SHG signals will occur only in 2D materials with a broken inversion symmetry [43] . Interestingly, the odd-numbered layers of PdSe 2 belong to the C 2h (2/m) point group and P2 1 /c (No.14) space group, which have an inversion symmetry, while the even-numbered layers possess a C 2v (mm2) point group and Pca2 1 (No. 29) space group with a broken inversion symmetry [23] . Meanwhile, the bulk PdSe 2 has an orthogonal structure with a D 2h point group and Pbca (No. 61) space group with an inversion symmetry [23] . These characteristics, that lead to the unique layer dependence of the SHG signal of PdSe 2 flakes, are very unlike that of the other 2D materials that have an inversion symmetry in the even layers and a broken inversion symmetry in the odd layers [42] , [44] . Additionally, it was found that the PdSe 2 samples were very uniform in thickness, attributing to the gold-assisted exfoliation method. Fig. 3: SHG spatial mapping of few-layer PdSe 2 . a , c The optical images of the PdSe 2 flakes for the SHG characterization. The red boxes indicate the selected area for the SHG measurements. The layer numbers are labeled by the white numbers. The region elected in a contain 1–5 L and 8 L PdSe 2, and the area selected in c includes 1–7 L PdSe 2 , ensuring sufficient sampling. The PdSe 2 samples were excited by 800 nm wavelength using 50× objective with a NA value of 0.55. b , d The spatial mapping of the integrated SHG signals corresponding to the regions in a and c , respectively. The intensities of the SHG signals are different for different layers. The SHG signal is almost absent in the odd-layer PdSe 2 , while it is strong in the even-layer PdSe 2 . The color bars are shown on the right of the figure. Full size image Generally, there are many factors that can influence the SHG intensity of PdSe 2 , and among those the excitation wavelength is relatively a significant one. To determine the wavelength that could generate the highest SHG signal, the SHG spectra were acquired by changing the excitation wavelengths from 780 to 1000 nm at a step length of 20 nm. As shown in Fig. 4a , there were strong excitation wavelength-dependent optical signals. The highest optical signal was observed under 880 nm excitation, which could be caused by the SHG effect. To explore the physical mechanism under excitation at 880 nm, the correlation between the detected optical intensity and the excitation intensity was measured. As presented in Fig. 4b , it was found that the optical intensity was quadratically dependent on the excitation power, and this was definitely the SHG signal. In addition, when excited with the same wavelength, the layer-dependent SHG signals of PdSe 2 were measured. As expected, the odd-numbered layers (1, 3, 5, and 7 L) exhibited very low SHG intensities while the even-numbered layers (2, 4, 6, and 8 L) displayed much stronger SHG signals. The SHG intensities as a function of the layer numbers were plotted in Fig. 4c , and it can be seen that the highest SHG intensity occurred in 4 L PdSe 2 (inset). The SHG intensity of PdSe 2 is mainly affected by two factors, the asymmetry and absorption intensity [28] , [45] . The odd-numbered layers of PdSe 2 (1, 3, 5, and 7 L) reserve the symmetry so that no distinct SHG signal is detected. However, as the layer number increased, the signal was weak and non-zero. This was due to the small but finite optical phase shift between the PdSe 2 layers [28] . Additionally, in the even-numbered layers (2, 4, 6, and 8 L) of PdSe 2 , as the layer number increased, the asymmetry of PdSe 2 increased, which caused a strong SHG signal in 4 L PdSe 2 [46] . However, when the layer number was more than 4 L, the optical absorption intensity in PdSe 2 became much stronger, leading to a lower collection efficiency of SHG [47] . Therefore, influenced by these two factors, the 4 L PdSe 2 exhibited the strongest SHG intensity. In general, the NLO process in a crystal can be expressed by the relationship of polarization vector and the electric field of the incident light in the form of [1] , [2] : 
    𝐏 = ε _0( χ𝐄 + χ ^( 2 )𝐄^2 + χ ^( 3 )𝐄^3 + ⋯)
 (1) where \({\mathbf{P}}\) is the polarization vector, and \(\varepsilon _0\) is the permittivity in a vacuum, while \(\chi\) is the electric susceptibility of the medium, and \({\mathbf{E}}\) is the electric field component of the incident light. For the SHG process, the dominated term is \({\mathbf{E}}^2\) . The second-order electric susceptibility, \(\chi ^{\left( 2 \right)}\) , reflects the SHG efficiency, and for 4 L PdSe 2, it was determined to be 5.17 × 10 −11 m V −1 at the excitation of 880 nm, according to Eqs. S1– 3 in the Supplementary Information (Note S1). The \(\chi ^{\left( 2 \right)}\) values for different 2D materials are presented in Table S1 . It can be seen that the \(\chi ^{\left( 2 \right)}\) value of PdSe 2 is comparable to that of the other 2D materials. Fig. 4: SHG characterization of the PdSe 2 flakes. a The SHG intensities excited at various wavelengths from 780 to 1000 nm, represented by different colors. The highest intensity appeared at the wavelength of 440 nm, manifesting the strongest SHG signal of excitation at 880 nm. b The excitation power dependence of SHG intensities in 4 L PdSe 2 . Both axes are shown on the log scale. The correlation of the pump power and SHG intensities exhibits was linear with a slope of 1.9 ± 0.12. c The SHG signal excited at the fixed wavelength of 880 nm in 1–8 L PdSe 2 . The integrated intensity of SHG varied with different layers, represented by the blue dots. The SHG signal was the strongest in the 4 L sample. The inset represents the SHG intensities versus the layer numbers of PdSe 2 . d The purple dots indicate the polar plot of integrated SHG intensities excited by the 880 nm laser in 4 L PdSe 2 . The corresponding fitting result is denoted by the solid red curve. Full size image Besides, the polarization-resolved SHG signals were also acquired, with the aim of identifying the crystal orientation of the sample. In our measurement, the polarization orientations of the incident and detected lights were parallel (for more specific information, see Experimental details). The experimental configuration and the measured parameters of the SHG measurement are illustrated in Fig. S3 in the Supplementary Information. Under a parallel configuration, the polar plot of the SHG signals represented distinct anisotropy, embodied in a dumbbell shape (Fig. 4d ). The SHG intensity had its minimum at 0°, then it gradually increased as the polarization orientation rotated, reaching the maximum at 90°. The slight skewing of the polar plot might be resulted from the distorted crystal lattice. The nonlinear dielectric susceptibility tensor was employed to analyze the polarization-resolved SHG signals. The SHG polarization vector, \({\mathbf{P}}\) , is related to the electrical field, \({\mathbf{E}}\) , of the incident light, and their relationship is expressed as [46] 
    𝐏 = d𝐄
 (2) where d is the dielectric susceptibility tensor. Under the three-dimensional geometric space, both \({\mathbf{P}}\) and \({\mathbf{E}}\) have three components in the x, y, and z directions. Likewise, other variables also have a three-dimensional form. Therefore, the above formula can be further expressed as follows 
    ( [ P_x; P_y; P_z ]) = ( [ [ d_11 d_12 d_13; d_21 d_22 d_23; d_31 d_32 d_33 ] [ d_14 d_15 d_16; d_24 d_25 d_26; d_34 d_35 d_36 ] ])( [    [ E_xE_x; E_yE_y; E_zE_z ]; [ 2E_yE_z; 2E_xE_z; 2E_xE_y ] ])
 (3) where d ij is the element of the dielectric susceptibility tensor. For the experimental backscattering setup, the electrical field intensity of the incident light in the z-direction was negligible. Thus, the electrical field intensities in the x and y directions can be expressed as 
    [ E_x = E_0cosθ; E_y = E_0sinθ ]
 (4) where \(E_0\) is the module of the electrical field intensity of the incident light, and \(\theta\) is the angle between the x -axis of the crystal lattice of PdSe 2 and the polarization orientation of the incident light. Under the parallel backscattering configuration, the eventual SHG intensity is only correlated with \(P_x\) and \(P_y\) , expressed as 
    I_∥∝( P_xcosθ + P_ysinθ)^2
 (5) where \(I_\parallel\) is the detected SHG intensity under the parallel configuration. Substitute Eq. ( 3 ) with Eq. ( 5 ), we obtained 
    I_∥∝[ [    d_11cosθ ^3 + ( d_21 + 2d_16)cosθ ^2sinθ; +  ( d_12 + 2d_26)cosθsinθ ^2 + d_22sinθ ^3 ]]^2
 (6) Using this formula, the experimental SHG intensities were fitted appropriately, as shown by the solid red curve in Fig. 4d . 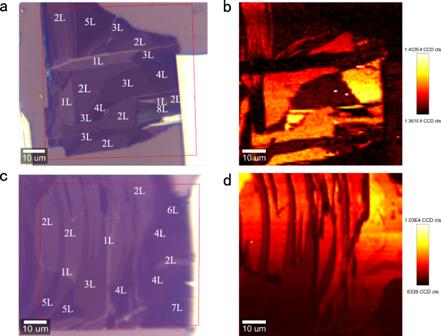Fig. 3: SHG spatial mapping of few-layer PdSe2. a,cThe optical images of the PdSe2flakes for the SHG characterization. The red boxes indicate the selected area for the SHG measurements. The layer numbers are labeled by the white numbers. The region elected inacontain 1–5 L and 8 L PdSe2,and the area selected incincludes 1–7 L PdSe2, ensuring sufficient sampling. The PdSe2samples were excited by 800 nm wavelength using 50× objective with a NA value of 0.55.b,dThe spatial mapping of the integrated SHG signals corresponding to the regions inaandc, respectively. The intensities of the SHG signals are different for different layers. The SHG signal is almost absent in the odd-layer PdSe2, while it is strong in the even-layer PdSe2. The color bars are shown on the right of the figure. It can be seen that the experimental results are entirely consistent with the theoretical analysis. 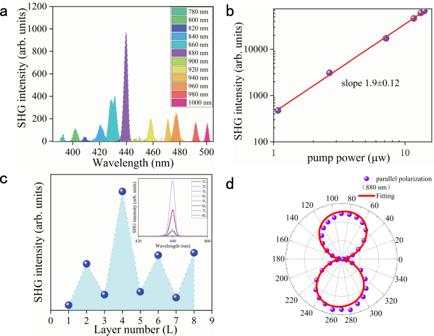Fig. 4: SHG characterization of the PdSe2flakes. aThe SHG intensities excited at various wavelengths from 780 to 1000 nm, represented by different colors. The highest intensity appeared at the wavelength of 440 nm, manifesting the strongest SHG signal of excitation at 880 nm.bThe excitation power dependence of SHG intensities in 4 L PdSe2. Both axes are shown on the log scale. The correlation of the pump power and SHG intensities exhibits was linear with a slope of 1.9 ± 0.12.cThe SHG signal excited at the fixed wavelength of 880 nm in 1–8 L PdSe2. The integrated intensity of SHG varied with different layers, represented by the blue dots. The SHG signal was the strongest in the 4 L sample. The inset represents the SHG intensities versus the layer numbers of PdSe2.dThe purple dots indicate the polar plot of integrated SHG intensities excited by the 880 nm laser in 4 L PdSe2. The corresponding fitting result is denoted by the solid red curve. Meanwhile, the polarization-resolved SHG measurements are expected to accurately identify the crystal orientation of PdSe 2 at the macro scale. TPA properties of PdSe 2 flakes The NLO processes in 2D materials can be divided into two classifications, the parametric and non-parametric process [48] . The parametric process in 2D materials is mainly a scattering process, where the ground state is excited into a virtual state, and there is no electron transfer and absorption between the two virtual states, such as the SHG above. On the contrary, the non-parametric process is the excitation from the ground state to a real state, which involves absorption and electron transfer, mainly including TPA and SA. To deeply explore the NLO properties of PdSe 2 , its TPA was further investigated. Figure S4 illustrates the experimental setting of the home-built nonlinear transmittance system used to perform the TPA and SA measurements, together with the measured parameters. To perform the TPA measurement, the monolayer and few-layer PdSe 2 flakes, obtained from the bulk crystal by gold-assisted exfoliation, were transferred to the transparent quartz substrates. After that, their TPAs were measured using the nonlinear transmittance method. According to our previous reports, PdSe 2 exhibits distinct linear dichroism features under the excitation of 300–800 nm [24] . When the excitation wavelength was 800 nm, the linear absorption coefficients of 1, 2, and 3 L PdSe 2 were estimated to be 3.9 × 10 3 , 1.3 × 10 4 and 1.9 × 10 4 cm −1 , respectively, according to the linear absorption measurement in Fig. S5 in Supplementary Information. Thus, the linear absorption was almost negligible in the solid film. Consequently, TPA could be predicted when excited by pulses at 800 nm. As intuitively described in Fig. 5 , the transmittance of the PdSe 2 flakes decreased with the increasing of the incident light intensity, exhibiting a typical TPA characteristic. Fig. 5: TPA properties of 1–3 L and bulk PdSe 2 flakes. a – c Nonlinear transmittance of 1–3 L PdSe 2 . The blue, green, and yellow dots represent the experimental data, while the solid red lines show the fitted results using the TPA model. The TPA coefficients ( β ) of 1, 2, and 3 L PdSe 2 are 4.16 × 10 5 , 2.58 × 10 5 , and 1.51 × 10 5 cm GW −1 , respectively. d Nonlinear transmittance of bulk PdSe 2 . The blue dots represent the experimental results, while the solid red lines show the fitted results using the TPA model. The TPA coefficient ( β ) of bulk PdSe 2 is 1.80 × 10 4 cm GW −1 . All the above measurements were performed under 800 nm excitation. Full size image Based on the nonlinear transmittance method, the TPA coefficients of the samples could be determined by the following formula [49] : 
    T( I_0) = I_t/I_0 = [ ln( 1 + I_0tβ)]/I_0tβ
 (7) where \(T(I_0)\) is the transmittance of the PdSe 2 sample, and \(I_{\mathrm{t}}\) is the transmitted light intensity of the sample, while \(I_0\) is the incident irradiance intensity and β is the TPA coefficient with \(t\) being the thickness of the PdSe 2 sample. By fitting the experimental data with Eq. ( 7 ), the β values of 1, 2, 3 L, and bulk PdSe 2 were determined to be 4.16 × 10 5 , 2.58 × 10 5 , 1.51 × 10 5 , and 1.80 × 10 4 cm GW −1 , respectively. These values are two to three orders of magnitude larger compared to those of other conventional semiconductors, such as MoS 2 , WS 2 , GaAs, CdS, and ZnO (Table S2 in Supplementary Information) [29] , [30] , [31] , [50] , meaning the great potential of the few-layer PdSe 2 flakes for TPA-based applications. Such giant TPA coefficients might originate from the strong exciton effects in PdSe 2 [51] . 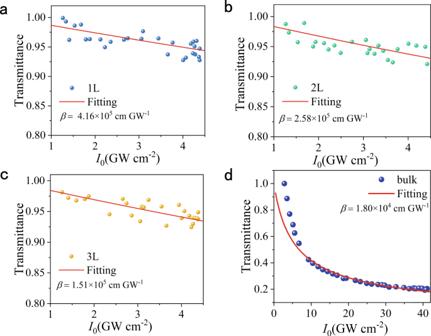Fig. 5: TPA properties of 1–3 L and bulk PdSe2flakes. a–cNonlinear transmittance of 1–3 L PdSe2. The blue, green, and yellow dots represent the experimental data, while the solid red lines show the fitted results using the TPA model. The TPA coefficients (β) of 1, 2, and 3 L PdSe2are 4.16 × 105, 2.58 × 105, and 1.51 × 105cm GW−1, respectively.dNonlinear transmittance of bulk PdSe2. The blue dots represent the experimental results, while the solid red lines show the fitted results using the TPA model. The TPA coefficient (β) of bulk PdSe2is 1.80 × 104cm GW−1. All the above measurements were performed under 800 nm excitation. This was enhanced by the strong dielectric screening owing to the ultrathin structure of the monolayer [23] , [52] . In addition, it was found that the TPA coefficient of PdSe 2 gradually decreased with the increasing of layers. Such a phenomenon was mainly attributed to the fact that the bandgap decreased with the increase of the number of layers, and there was a certain detuning between the formative exciton and the two-photon energy [53] . SA properties of PdSe 2 flakes Considering that strong SA was widely reported in various two-dimensional TMDCs, including MoS 2 [54] , WS 2 [55] , WSe 2 [56] , and MoSe 2 [57] , a typical SA effect could also be expected in our PdSe 2 in the case of 600 nm excitation. 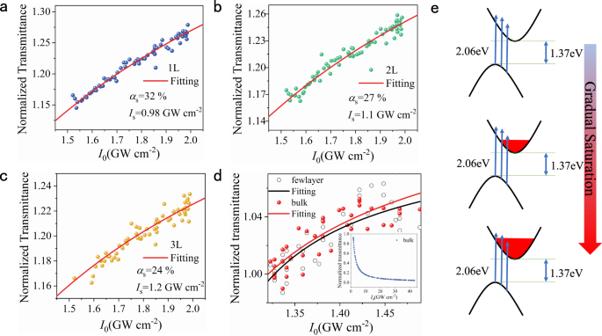Fig. 6: SA properties of 1–3 L and bulk PdSe2flakes. a–cNonlinear transmittance of 1–3 L PdSe2. The blue, green, and yellow dots represent the experimental data, while the solid red lines show the fitted results using the SA model. The SA intensities of 1, 2, and 3 L PdSe2are 0.98, 1.1, and 1.2 GW cm−2, respectively. The modulation depths of 1, 2, and 3 L PdSe2are 32%, 27%, and 24%, respectively.dNonlinear transmittance of the bulk PdSe2. The white and red dots represent the experimental data, while the black and red solid lines show the fitting curves of few-layer and bulk PdSe2using the SA model. The inset shows a reverse SA trend of the thick bulk PdSe2with increased laser power.eThe electronic transition process of SA. All the above measurements were performed under 600 nm excitation. Figure 6 shows the trends of the normalized transmittance versus the incident intensity in 1–3 L and bulk PdSe 2 . The fitting could be performed according to a standard model of SA, as shown in the following formula [58] : 
    T( I_0) = 1 - α _s/1 + I_0/I_s - α _u
 (8) where \(\alpha _{\mathrm{s}}\) is the modulation depth, and \(I_{\mathrm{s}}\) is the saturable intensity, while \(\alpha _{\mathrm{u}}\) is the unsaturated absorption component. The obtained fitting parameters of the modulation depths ( α s ) of 1–3 L PdSe 2 were 32%, 27% and 24%, respectively. The saturable intensities (usually the half of the highest optical absorption) of 1–3 L PdSe 2 were 0.98, 1.1, and 1.2 GW cm −2 , respectively. As the sample thickened, the saturable intensity gradually increased. The modulation depths are much higher than that of the most other 2D materials, such as SnSe [32] , MoSe 2 [33] , MoS 2 [34] , and PtSe 2 [59] , which are promising for the application in ultrafast lasers. The high modulation depths mainly resulted from the low unsaturated loss, indicating a low defect density in the PdSe 2 [7] . However, the modulation depths in (thinner) bulk and few-layer PdSe 2 (more than 10 L, only 2.8%) were much lower than that in 1–3 L PdSe 2 , which might be attributed to the increased unsaturated loss induced by the strengthened scattering [7] . It is worth noting that there was no SA phenomenon for the thicker bulk PdSe 2 since when the sample was thick enough, the light capacity was sufficient, and the saturation state would not be easily reached. The excellent SA property of 1–3 L PdSe 2 endows its application prospect in the field of ultrafast lasers. Fig. 6: SA properties of 1–3 L and bulk PdSe 2 flakes. a – c Nonlinear transmittance of 1–3 L PdSe 2 . The blue, green, and yellow dots represent the experimental data, while the solid red lines show the fitted results using the SA model. The SA intensities of 1, 2, and 3 L PdSe 2 are 0.98, 1.1, and 1.2 GW cm −2 , respectively. The modulation depths of 1, 2, and 3 L PdSe 2 are 32%, 27%, and 24%, respectively. d Nonlinear transmittance of the bulk PdSe 2 . The white and red dots represent the experimental data, while the black and red solid lines show the fitting curves of few-layer and bulk PdSe 2 using the SA model. The inset shows a reverse SA trend of the thick bulk PdSe 2 with increased laser power. e The electronic transition process of SA. All the above measurements were performed under 600 nm excitation. Full size image To understand the principle of the transmittance dependence on the incident irradiance, the electronic transition process in the momentum space should be clear. Figure 6e illustrates the electronic transition process of SA in PdSe 2 . The bandgap of the monolayer (bulk) PdSe 2 was determined to be 1.37 (0.03) eV (Fig. S6 in Supplementary Information), indicating the unusual indirect bandgap characteristics. In our case, the energy of the incident photon (2.06 eV) was much higher than the bandgap of a few-layer PdSe 2 . For low excitation intensity, the electrons in the valence band jumped to the relatively high energy levels in the conduction band, as illustrated on the top panel of Fig. 6e . Then, the hot electrons relaxed to the lower energy band, and populated in the bottom of the conduction band. With the increase in incident optical intensity, the number of excited electrons also increased. Electron is a fermion, that cannot populate at the same energy level. Thus, the energy levels were gradually filled from the bottom to the top in the conduction band (middle panel in Fig. 6e ). When the energy level of the conduction band was filled with electrons as the incident light intensity increased, the electronic transition process was impeded owing to the Pauli exclusion principle. The number of the absorbed photons then gradually approached saturation, as indicated on the bottom panel of Fig. 6e . This explains the gradually saturable transmittance when the incident optical intensity was progressively increased. In summary, large-area PdSe 2 flakes with different thicknesses were successfully fabricated on the Si/SiO 2 and quartz substrates. Significantly, in contrast to that of the other 2D materials, robust broadband SHG properties in the even-numbered layers of PdSe 2 were demonstrated, as a result of the unique anisotropic puckered pentagonal structure of PdSe 2 . Besides, the TPA and SA characteristics of the PdSe 2 flakes were investigated. Under the excitation at 800 nm, 1–3 L and bulk PdSe 2 exhibited giant TPA coefficients ( β ) of 4.16 × 10 5 , 2.58 × 10 5 , 1.51 × 10 5 , and 1.80 × 10 4 cm GW −1 , respectively, which are at least two orders of magnitude larger than those of the conventional semiconductors. Interestingly, when the excitation was switched to 600 nm, on account of the ultra-low unsaturable loss, strong SA with the modulation depths ( α s ) up to 32%, 27% and 24% for 1–3 L PdSe 2 were observed. Compared to those of the other traditional 2D materials, these values are exceptionally large. Such prominent NLO activity of 2D PdSe 2 provides great prospects for potential applications in optical switching, ultrafast lasers, saturation absorbers, optical limiters, and micro/nano optical modulation devices. Sample preparation The PdSe 2 flakes were exfoliated from bulk single-crystal PdSe 2 (HQ graphene) onto silicon and transparent quartz substrates, employing the gold-assisted exfoliation. The thicknesses of the 1, 2, 3 L, and bulk PdSe 2 were 0.7, 1.4, 2.1, and 10.5 nm, respectively. Raman single-spectrum characterization A WITec Alpha 300 R was utilized to obtain the high-resolution spectra. A 532 nm laser was used to excite the PdSe 2 flakes with a power of 0.25 mW, a 100× objective with NA = 0.9, and a laser spot size of 1 μm. The integration time was 5 s with accumulated ten times to obtain a high signal-to-noise ratio. The 1800 g mm −1 optical grating was used to improve the spectral resolution. SHG measurements and characterization The reflective geometry with normal incidence excitation was used to achieve the SHG measurements. The ultrashort 80 fs pulses with a 80 MHz repetition rate (Spectra-Physics Solstice Maitai HP) were used as the excitation source for the SHG measurements. For SHG mapping characterization, the regions of 40 × 40 μm 2 and 50 × 50 μm 2 containing 1–8 L PdSe 2 flakes were selected. A fiber-based pulsed laser was used as the fundamental pump source with the center wavelength at 800 nm. The laser pulses were focused onto a spot size of 6 μm on the PdSe 2 sample by a 50× objective with NA = 0.55. The same objective lens was used to collect the SHG signal scattered from the sample and then detected by the charged coupling device (CCD) spectrometer. The integration time of 0.5 s and the scan duration of 2 h was set to achieve the high-resolution mapping images. For the measurements of layer number dependent SHG signal, the excitation wavelength was fixed at 880 nm, and the same excitation intensity was used. For SHG polarization measurements, a half-wave plate (analyzer) was placed in the incident (outgoing) light path. Only the light with its polarization orientation parallel to the optical axis of the analyzer could pass and be detected by the CCD spectrometer. A step size of 10° was adopted for the parallel configuration. TPA and SA measurements The TPA and SA of PdSe 2 were measured using the nonlinear transmittance method in a home-built micro NLO system.The samples were excited at the wavelength of 600 nm (spectral width ~15 nm) or 800 nm (spectral width ~10 nm) by the laser pulses from an OPA combined with TOPAS (1000 Hz, 110 fs, Spectra-Physics, Inc.). The fs pulses were focused onto the sample by A 50× objective lens with NA = 0.55.